Ligand-enabled Ni-catalysed enantioconvergent intermolecular Alkyl-Alkyl cross-coupling between distinct Alkyl halides α-Tertiary aliphatic amides are key elements in organic molecules, which are abundantly present in natural products, pharmaceuticals, agrochemicals, and functional organic materials. Enantioconvergent alkyl-alkyl bond-forming process is one of the most straightforward and efficient, yet highly challenging ways to build such stereogenic carbon centers. Herein, we report an enantioselective alkyl-alkyl cross-coupling between two different alkyl electrophiles to access α-tertiary aliphatic amides. With a newly-developed chiral tridentate ligand, two distinct alkyl halides were successfully cross-coupled together to forge an alkyl-alkyl bond enantioselectively under reductive conditions. Mechanistic investigations reveal that one alkyl halides exclusively undergo oxidative addition with nickel versus in-situ formation of alkyl zinc reagents from the other alkyl halides, rendering formal reductive alkyl-alkyl cross-coupling from easily available alkyl electrophiles without preformation of organometallic reagents. α-Tertiary aliphatic amides with a α-saturated stereogenic carbon center are key structural units in chemistry, functional materials and many related areas [1] , [2] , [3] , [4] , [5] . Thus, the development of versatile and straightforward methods to access saturated stereogenic centers in a highly enantioenriched manner has been attracting long-term interests from chemistry community [6] . Early efforts have been paid to the employing of chiral auxiliaries to control the desired stereochemistry, resulting in the use of stoichiometric amount of chiral auxiliaries as well as additional steps for their installation and removal from the target molecules [7] . Over the past decades, studies have been increasingly focused on catalytic approaches to access such stereogenic centers [8] , [9] , including Ni-catalysed enantioconvergent cross-coupling between an alkyl electrophile and an alkyl nucleophile (Fig. 1a ) [10] , [11] . Over the past years, significant progress has been achieved in nickel-catalysed enantioselective cross-coupling of racemic secondary alkyl electrophiles with organometallic reagents [12] , [13] , [14] , [15] , [16] , [17] , [18] , [19] , [20] . This reaction mode has been well-developed and evolved into an inevitable tool for constructing saturated stereogenic carbon centers. Although the significant advances, this reaction mode requires stoichiometric, reactive, and often sensitive organometallic reagents, which usually require time-consuming preformation. To this end, one alternative is to use alkenes as masked alkyl nucleophiles in the presence of metal hydride to undergo enantioselective alkyl-alkyl cross-coupling [21] , [22] , [23] , [24] . Hydrometallation of alkenes through metal hydride insertion generates alkyl metallic intermediates in situ as alkyl nucleophiles. In 2019, Fu group reported a seminal work on Ni-H catalysed enantioselective alkyl-alkyl cross-couplings of 1-substituted alkenes as a surrogate of carbon nucleophile to couple with secondary alkyl bromides adjacent to amides and esters (Fig. 1b ) [25] , [26] . More recently, secondary alkyl bromides next to phosphates and ethers were successfully involved [27] , [28] , [29] , [30] , [31] , [32] , [33] . Accordingly, this strategy has evolved into an efficient cross-coupling of diverse alkenes with alkyl electrophiles to build saturated stereogenic carbon centers in the presence of metal hydrides [34] , [35] . Fig. 1: Strategies for intermolecular enantioselective construction of alkyl-alkyl bonds. a Enantioselective C sp3 -C sp3 bond-forming from alkyl-M and alkyl electrophiles. b Enantioselective C sp3 -C sp3 bond-forming from alkenes and alkyl electrophiles. c Enantioselective C sp3 -C sp3 bond-forming from two alkyl electrophiles. Full size image However, direct reductive cross-coupling between two distinct electrophiles is still one of the most straightforward, cost-effective, thus ideal alternatives to construct saturated stereogenic carbon centers [36] , [37] , [38] . Ni-catalysed cross-coupling reactions between organ-electrophiles under reductive conditions have been extensively investigated for C sp2 -C sp3 bond formation [39] , [40] , [41] , [42] , [43] , [44] . To date, no example of non-enzyme-catalysed enantioselective C sp3 -C sp3 bond formation was reported [45] . Herein, we report a Ni-catalysed intermolecular cross-coupling between two different alkyl electrophiles under reductive conditions (Fig. 1c ). The use of newly-developed chiral ligand enables construction of C sp3 -C sp3 bond by selective coupling of two distinct alkyl electrophiles, without the preformation of organometallic reagents. Optimization of the reaction conditions To prove the concept, we commenced the investigation using 1a and 2a as the prototype substrates using nickel catalysis to evaluate the reaction parameters. After extensive preliminary evaluation (See Supplementary Tables 1 – 5 ), we found the use of pyridine-BOX type ligands gave better results compared to other types of ligands in the presence of zinc (3.0 equiv) as sacrificing reductant, ferrous chloride (25 mol%), and cesium iodide (3.0 equiv) as additives. 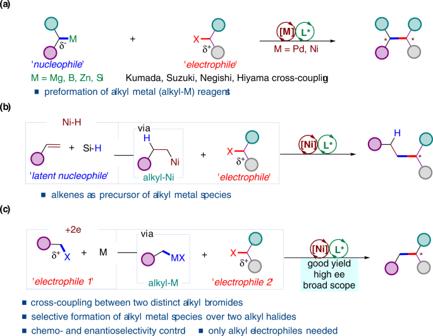Fig. 1: Strategies for intermolecular enantioselective construction of alkyl-alkyl bonds. aEnantioselective Csp3-Csp3bond-forming from alkyl-M and alkyl electrophiles.bEnantioselective Csp3-Csp3bond-forming from alkenes and alkyl electrophiles.cEnantioselective Csp3-Csp3bond-forming from two alkyl electrophiles. Among the tested known ligands, L1 gave the best result, delivering the desired cross-electrophile coupling product 3a in 67% yield with 70% ee (Table 1 , entry 1). Modifying the substituents at α-position to oxygen on the oxazolidine ring of i Pr-PyBOX significantly altered the efficiency of the ligand for this reaction (Table 1 , entries 2–7). Linear substituents at α-position to oxygen of i Pr-PyBOX ( L2 - L4 ) substantially diminished the yield and enantioselectivity (Table 1 , entries 2–4). Cyclic substituents slightly increased the enantioselectivity of 3a from 70% to 76% and 71%, respectively (Table 1 , entries 5 and 6). Introducing two phenyl groups onto α-position to oxygen ( L7 ) led to trace amount of 3a (Table 1 , entry 7). Next, Bn-PyBOX derived ligands ( L8 - L12 ) were applied to this asymmetric cross-electrophile coupling reaction (Table 1 , entries 8-12). Bn-PyBOX delivered the desired product 3a in 29% yield with 60% ee (Table 1 , entry 8). Increasing the steric hindrance at the α-position to oxygen improved the enantiomeric excess of 3a to 84% (Table 1 , entry 10). Ligands derived from i Bu-PyBOX ( L13 - L15 ) gave inferior yields and enantioselectivity (Table 1 , entries 13-15). When Et-PyBOX based ligand L16 was used, 3a was obtained in 29% yield with 90% ee (Table 1 , entry 16). Then, Me-PyBOX derived ligands ( L17 - L23 ) were tested (Table 1 , entries 17-23). The use of propyl Me-PyBOX ( L20 ) furnished 3a in 21% yield with 94% ee (Table 1 , entry 20). Further evaluation of additive and solvent effect revealed that the addition of 15-crown-5 (10 mol%) in a mixture of DMA and diglyme (1:3) afforded 3a in 85% yield with 94% ee (See Supplementary Tables, 7 - 11 ). The use of ferrous chloride may facilitate the cross-coupling of 1a with 2a . In addition, the addition of 15-crown-5 may serve as an additive to enhance the solubility of inorganic salts in organic phase. Table 1 Ligand effect on the enantioselective formal reductive alkyl-alkyl cross-coupling reaction a Full size table Scope of the reaction With the optimized conditions in hand, we turned to test the scope of this reaction (Figs. 2 and 3 ). First, we examined the viability of α -bromoamides 1 (Fig. 2 ). Various substituted aniline derived α -bromoamides were good substrates for this enantioselective cross-electrophile alkyl-alkyl coupling reaction ( 3b - 3r ). Electron-donating group substituted aniline based amides delivered the desired enantioenriched α -alkylated amides in 58%–67% yields with 88–94% ee ( 3b - 3e ). Electron-withdrawing groups were also tolerated in the reaction, delivering the corresponding α -tertiary amides in 51–73% yields with 93–94% ee ( 3f - 3k ). Ketones and esters were compatible under the reaction conditions, giving the ketone and ester containing α -tertiary amides in 60% and 71% yields with 93% ee ( 3g - 3h ). Halides, such as fluorine, chlorine, and bromine, were also well-tolerated in this nickel-catalysed reductive process ( 3i - 3k ), leaving halides as a chemical handle for further elaboration. Notably, free phenol was tolerated in the catalytic process, furnishing desired enantioenriched amide 3 l in 51% yield with 91% ee. Moreover, meta- and ortho- substituted as well as 2-naphthylamine derived α-bromoamides could be converted to corresponding α-alkylated amides in 58–71% yields with 92–94% ee ( 3m-3q ). Thiophene amine was tolerated in the reaction, giving the desired product 3r in 67% yield with 94% ee. Aliphatic amines, including the linear, branched, and benzylic amine based α-bromoamides were all good substrates, giving the desired products in synthetic useful yields with 82–88% ee ( 3s-3v ). α-Bromoamide from chiral amine was converted to α-alkylated amide 3w in 63% yield with 9:1 dr. Impressively, unprotected α-bromoamides, which are challenging for enantioselective coupling reactions, could be tolerated to deliver corresponding reductive cross alkyl-alkyl coupling product 3x in 49% yield with 87% ee. In addition, α-bromo- N , N -disubstituted amide is applicable in this reaction, affording the cross-coupling product ( 3y ) in 52% yield with 92% ee. Unfortunately, α-bromo ester failed to deliver the desired cross-coupling product ( 3z ) under the reaction conditions. Next, we embarked to test the scope of α-substituent of amides. Diverse alkyl substituents with different chain length were good substrates, delivering corresponding α-alkylated amides ( 4a and 4b ) in 69% and 65% yields with 94% ee, respectively. Notably, α-chloroamides successfully underwent asymmetric alkyl-alkyl cross-coupling with 2a to give 4a in 61% yield with 92% ee. More steric demanding substituents, such as isopropyl, cyclopentylmethyl were also compatible in the reaction, giving 4c and 4d in 50% and 63% yields with 89% and 90% ee. Benzyl, phenylethyl, chloroethyl, and allyl could be tolerated in the reaction, giving the desired products 4e-4h in 58%-67% yields with 91%-92% ee. Notably, the enantioenriched amides with similar steric hindrance at α-position could be achieved with excellent enantioselectivity ( 4f ). The absolute configuration of the product was further confirmed by the X-ray diffraction analysis of 4f . Fig. 2: Scope of α -bromoamides. The reaction was performed on a 0.2 mmol scale under the conditions in Table 1 , entry 24. 15C5 = 15-crown-5. DME dimethoxyethane, DMA dimethylacetamide. 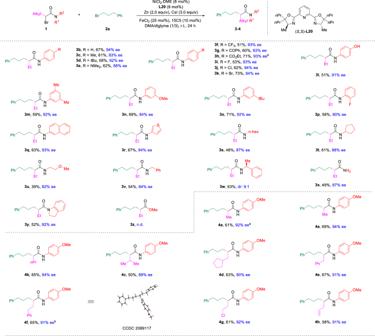Fig. 2: Scope ofα-bromoamides. The reaction was performed on a 0.2 mmol scale under the conditions in Table1, entry 24. 15C5 = 15-crown-5. DME dimethoxyethane, DMA dimethylacetamide. Note:aα-Chloroamide was used instead ofα-bromoamide.b3-Phenyl-1-iodopropane was used instead of2a. Note: a α -Chloroamide was used instead of α -bromoamide. b 3-Phenyl-1-iodopropane was used instead of 2a . Full size image Fig. 3: Scope of alkyl halides. The reaction was performed on 0.2 mmol scale under the conditions in Table 1 , entry 24. 15C5 = 15-crown-5. DME dimethoxyethane, DMA dimethylacetamide. Full size image Next, the scope of the other alkyl electrophile was evaluated (Fig. 3 ). Different alkyl bromides were good substrates for this enantioselective cross-electrophile coupling reaction, giving corresponding alkyl-alkyl products ( 5a - 5c ) in 47–66% yields with 89–92% ee. Many functional groups, such as chlorine, nitrile, amide, alkene, alkyne, acetal, ester, ether containing alkyl bromides could be coupled to deliver desired products in moderate to good yields with 90–94% ee ( 5d - 5m ). Heterocycles, such as thiophene and furan substituted alkyl halides were transformed into corresponding products ( 5n and 5o ) in 65% and 62% yields with 90% and 93% ee, respectively. Unfortunately, secondary unactivated alkyl halides remain unsuccessful for the reaction. In addition, both isomers of 6 were obtained under identical reaction conditions with the same chiral ligand. In the presence of ( S , S )- L20 , the reaction of 1a with 1-iodopropane gave R - 6 in 70% yield with 86% ee, while the reaction of 1b with ethyl bromide furnished the other isomer S - 6 in 59% yield with 88% ee. Mechanistic study In order to gain insight into the mechanism of the reaction, we set up a series of reactions to shed light on the reaction pathways (Fig. 4 ). First, the reaction of 1a with 2a in the presence of a radical scavenger TEMPO under otherwise identical to standard conditions was conducted (Fig. 4a ). The desired intermolecular cross-coupling product 3a was not formed. Instead, the adduct 7 of TEMPO with 1a was obtained in 85% yield, indicating α-bromoamides underwent a single electron transfer process in this transformation. Next, the reactions of alkyl bromides with preformed alkyl zinc reagents under the standard conditions were tested (Fig. 4b ). When alkyl zinc reagent 8 was used instead of 1a to couple with 2a under standard conditions, no desired product 3a was detected, and only protonated product 8’ was formed quantitatively, indicating alkyl zinc reagent 8 could not mediate the reaction under the standard reaction conditions. In contrast, the reaction of 1a with alkyl zinc reagent 9 under standard conditions delivered the desired cross-coupling product 3a in 87% yield with 89% ee. Further conducting the reaction with slow addition of alkyl zinc reagent 9 led to the formation of 3a in 83% yield with 94% ee, which is identical to the standard reaction conditions. These results suggest slow formation of alkyl zinc intermediate 9 in-situ to serve as intermediate for the reaction. To further prove the formation of alkyl zinc intermediates during the reaction, a real-time reaction course was conducted (Fig. 4c ). The monitor the reaction process of 1a with 2a under standard conditions showed that no formation of 3a in the first 30 min, although the consumption of 2a was observed, indicating the induction time to form significant amount of alkyl intermediate to initiate the coupling reaction to generate 3a . Fig. 4: Control experiments and mechanistic investigations. a Quench of radical intermediates. TEMPO tetramethylpiperidine oxide. b Reactions with alkyl zinc reagents. c Time course for 2a and 3a under standard conditions. Full size image On the basis of experimental results and literature precedence [46] , [47] , [48] , a plausible mechanism is depicted in Fig. 5 . First, Ni(II) was reduced by zinc to generate the ligated nickel (I) species ( Int-A ) in the presence of chiral ligand ( L ), which could undergo single electron transfer to 1 to give alkyl radical intermediate Int-B and Ni (II) intermediate Int-C . In the meantime, alkyl zinc reagent Int-D could be formed from 2 and zinc in the assistance with iodide, which could undergo transmetalation with Int-C to generate alkyl Ni(II) species Int-E . The rebound of intermediates Int-B and Int-E could form dialkyl Ni (III) intermediate Int-F , which would facilitate reductive elimination to furnish the final product 3 and regenerate Ni (I) species. 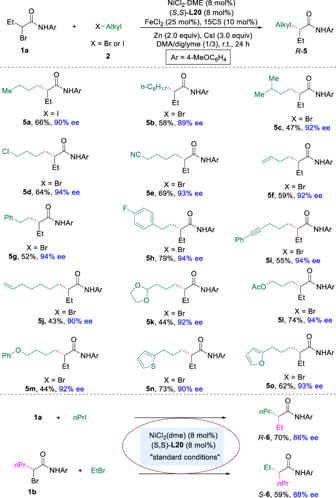Fig. 3: Scope of alkyl halides. The reaction was performed on 0.2 mmol scale under the conditions in Table1, entry 24. 15C5 = 15-crown-5. DME dimethoxyethane, DMA dimethylacetamide. Fig. 5: Proposed mechanism for the reaction. A plausible reaction mechanism for the intermolecular alkyl-alkyl cross-coupling between distinct alkyl halides based on all experimental results and previous literature evidence. Full size image In summary, an intermolecular enantioselective alkyl-alkyl cross-coupling between two alkyl electrophiles has been developed enabled by the efficient and selective cross-coupling reaction between two distinct alkyl halides under reductive conditions, representing an alternative for the construction of chiral C sp3 -C sp3 bonds. 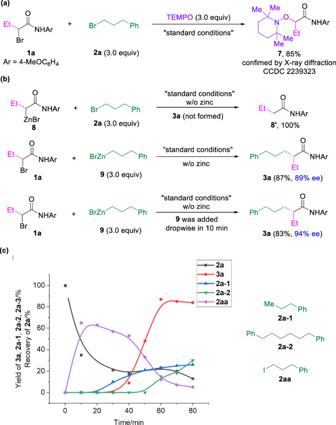Fig. 4: Control experiments and mechanistic investigations. aQuench of radical intermediates. TEMPO tetramethylpiperidine oxide.bReactions with alkyl zinc reagents.cTime course for2aand3aunder standard conditions. 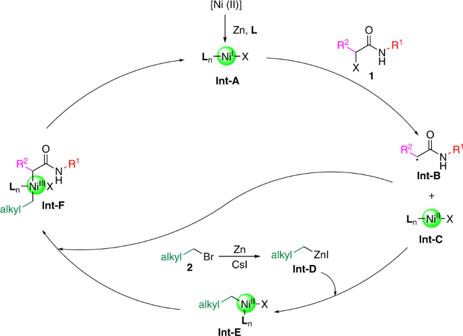Fig. 5: Proposed mechanism for the reaction. A plausible reaction mechanism for the intermolecular alkyl-alkyl cross-coupling between distinct alkyl halides based on all experimental results and previous literature evidence. One alkyl halides in-situ formed alkyl nucleophiles with reducing metal to cross-couple with the other alkyl halides in a chemo- and enantioselective manner, circumventing the tedious and time-consuming preformation of alkyl metal species. We anticipate this will inspire enantioselective in-situ cross-coupling between alkyl electrophiles under reductive conditions to be evolved into one of the major strategies to build saturated carbon centers via enantioselective C sp3 -C sp3 bond-formation. General procedure for Ni-catalysed enantioconvergent intermolecular alkyl-alkyl cross-coupling In a nitrogen-filled glovebox, NiCl 2 · glyme (0.016 mmol, 8 mol%), chiral ligand L20 (0.016 mmol, 8 mol%) and diglyme (1.0 mL) were added to a 10-mL vial equipped with a stir bar. The mixture was allowed to stir for 1 h, after which it was an orange solution. Then, FeCl 2 (0.05 mmol, 25 mol%), 15C5 (0.02 mmol, 10 mol%), CsI (0.6 mmol, 300 mol%), Zn (0.4 mmol, 200 mol%), 1 (0.2 mmol), 2 (0.6 mmol, 300 mol%), DMA (0.5 mL) and diglyme (0.5 mL) were added. The reaction mixture was transferred out of the glovebox and stirred (~1400 rpm) at room temperature for 24 h. Next, ethyl acetate (20.0 mL) was added, and the mixture was washed with water (10.0 mL) and brine (10.0 mL), dried over Na 2 SO 4 , filtered, and concentrated under vacuum. The residue was purified by flash chromatography on silica gel to afford the enantioselective alkyl-alkyl cross-coupling product.